Sub-50-nm self-assembled nanotextures for enhanced broadband antireflection in silicon solar cells Materials providing broadband light antireflection have applications as highly transparent window coatings, military camouflage, and coatings for efficiently coupling light into solar cells and out of light-emitting diodes. In this work, densely packed silicon nanotextures with feature sizes smaller than 50 nm enhance the broadband antireflection compared with that predicted by their geometry alone. A significant fraction of the nanotexture volume comprises a surface layer whose optical properties differ substantially from those of the bulk, providing the key to improved performance. The nanotexture reflectivity is quantitatively well-modelled after accounting for both its profile and changes in refractive index at the surface. We employ block copolymer self-assembly for precise and tunable nanotexture design in the range of ~10–70 nm across macroscopic solar cell areas. Implementing this efficient antireflection approach in crystalline silicon solar cells significantly betters the performance gain compared with an optimized, planar antireflection coating. Proper design of an antireflection coating involves managing the refractive index mismatch at the abrupt optical interface [1] . The most straightforward approach places a single layer of intermediate optical index at the interface to create destructive interference in the reflected light, providing full antireflection at a single wavelength, λ =4 n i · t , with material thickness ( t ) and refractive index , where n S and n A are the refractive indices of the substrate and air, respectively. Increasing broadband coverage, for application in transparent window coatings [2] , [3] , [4] , [5] , military camouflage [6] or solar cells [7] , [8] , [9] , [10] , [11] , [12] , [13] , [14] , [15] , is possible using thin-film multilayer schemes [16] . An alternative to thin-film-coating strategies instead patterns the interface at subwavelength dimensions, creating an effective medium between the substrate and air, with n i changing gradually from n A to n S [10] , [11] , [17] . Such structures, often called moth eyes because of their biomimicry, provide broadband antireflection over a wide range of incident light angles when subwavelength textures are taller than t ~0.4· λ and spaced closer than ℓ~ λ /2 n s [12] , [14] , [18] , [19] , [20] . In this work, we enhance the broadband antireflection properties of a nanofabricated moth eye structure through simultaneous control of both the geometry and optical properties, by designing nanotextures sufficiently small to take advantage of a beneficial material surface layer only a few nm thick. Nanotexture fabrication We leverage block copolymer self-assembly and plasma etching to fabricate highly regular surface nanotextures, with precise control over the texture’s lateral feature size in the range of 10–70 nm, vertical profile and feature density. Self-assembly based nanofabrication provides a scalable approach to creating deeply subwavelength moth eye structures (schematics in Fig. 1a ). We pattern surface nanotextures on polished (100) silicon by first self-assembling a cylindrical phase polystyrene-block-poly(methyl methacrylate) (PS- b -PMMA) block copolymer thin film ( M w =99 kg mol −1 , PS:PMMA ~7:3) by spin-coating and thermal annealing. Appropriate surface pretreatment facilitates perpendicular orientation of uniformly sized 25-nm-diameter PMMA cylindrical microdomains within a PS matrix, locally hexagonally arranged with a separation ℓ=52±6 nm [21] . We systematically vary ℓ in the nanotexture from 40±3 to 67±13 nm using block copolymers with total molecular weight ranging between 67 and 177 kg mol −1 . Exposing assembled copolymer films to three sequential cycles of tri(methyl aluminium) and water vapour selectively loads PMMA microdomains with alumina by sequential infiltration synthesis ( Fig. 1b ; Supplementary Fig. 1 ) [22] . 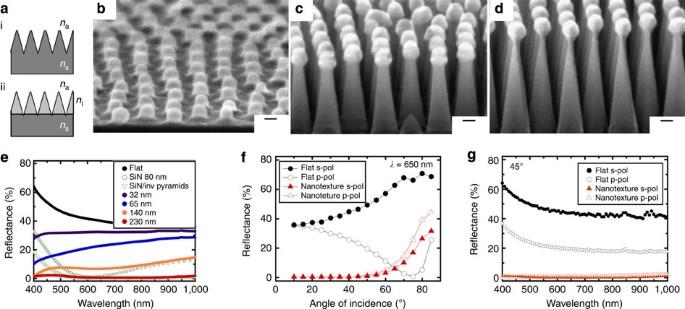Figure 1: Silicon nanotexture fabrication and optical reflectance. (a) Schematic (i) tapered antireflection nanotexture and (ii) tapered nanotexture with graded refractive index. (b) 70° Angle cross-sectional scanning electron microscope (SEM) image of close-packed alumina nanostructures formed by infiltrating a 99kg-mol−1cylindrical phase polystyrene-b-poly(methyl methacrylate) block copolymer. Scale bar, 20 nm. (c,d) 70° Angle cross-sectional SEM images of nanotextures fabricated by (c) 60 s and (d) 100 s of plasma etch. Scale bar, 20 nm. (e) Measured reflectance versusλfor a flat Si film, an 80-nm-thick silicon nitride film and nanotextures with ℓ=52 nm andtranging from 32 to 230 nm. Also shown is the simulated reflectance of an 80-nm-thick silicon nitride film on chemically etched inverted pyramids. (f) Measured reflectance (at 650 nm) for s- and p-polarization versus incident angle for flat silicon (black circles) and nanotextures with ℓ=52 nm andt=230 nm (red triangles). (g) Measured reflectance of s- and p-polarization versusλ(45° incident angle) for nanotextures with ℓ=52 nm andt=230 nm height. Figure 1: Silicon nanotexture fabrication and optical reflectance. ( a ) Schematic (i) tapered antireflection nanotexture and (ii) tapered nanotexture with graded refractive index. ( b ) 70° Angle cross-sectional scanning electron microscope (SEM) image of close-packed alumina nanostructures formed by infiltrating a 99kg-mol −1 cylindrical phase polystyrene- b -poly(methyl methacrylate) block copolymer. Scale bar, 20 nm. ( c , d ) 70° Angle cross-sectional SEM images of nanotextures fabricated by ( c ) 60 s and ( d ) 100 s of plasma etch. Scale bar, 20 nm. ( e ) Measured reflectance versus λ for a flat Si film, an 80-nm-thick silicon nitride film and nanotextures with ℓ=52 nm and t ranging from 32 to 230 nm. Also shown is the simulated reflectance of an 80-nm-thick silicon nitride film on chemically etched inverted pyramids. ( f ) Measured reflectance (at 650 nm) for s- and p-polarization versus incident angle for flat silicon (black circles) and nanotextures with ℓ=52 nm and t =230 nm (red triangles). ( g ) Measured reflectance of s- and p-polarization versus λ (45° incident angle) for nanotextures with ℓ=52 nm and t =230 nm height. Full size image The self-assembled alumina pattern provides a rugged template for creating surface nanotextures using plasma etching. We anisotropically etch the underlying silicon by inductively coupled plasma-reactive ion etching using a gas chemistry of hydrogen bromide, chlorine and oxygen, which produces a sidewall angle of >80° ( Fig. 1c,d ). The gas mixture and etch parameters control the nanotexture profile, with t increasing with etch time and taller nanotextures tapering to smaller sizes at their tops ( Fig. 1c,d ). Block copolymer self-assembly provides a scalable method for producing these controlled nanotextures over arbitrarily large areas, evidenced by its successful prior integration into 300-mm-diameter semiconductor wafer-processing facilities [23] . Previous investigations have used different block copolymer phases [5] , [24] and micelles [25] with larger length scales (>100 nm) as templates for nanotextures imparting antireflection to glass and silicon surfaces, which are too large to observe the enhancements described here. Nanotexture reflectance The average reflectance of the nanotextured silicon surface decreases with increasing feature height ( t ) in the λ range of 400 nm to 1 μ, from 35% on a flat surface to <1% for tapered nanotextures with t =230 nm and ℓ=52 nm ( Fig. 1e ). The nanotextured surface is significantly less reflective than antireflection methods employed in commercial silicon solar cells, including flat silicon coated with an 80-nm-thick silicon nitride layer ( Fig. 1e , green open circles) and chemically etched, inverted pyramid coatings ( Fig. 1e , green inverted triangles, simulated using OPAL 2 (ref. 26 )). This latter scheme requires sacrificing ~10 μ of silicon at the device top surface, which may have consequences for thin-film devices. In practice, all types of silicon solar cells are bonded to a protective glass or plastic top coating. In principle, block copolymer antireflection schemes can be applied to glass surfaces as well. The tapered vertical profile gradually changes n i from air ( n A =1) to silicon ( n S =5.6 at 400 nm; n S =3.6 at 1 μm). Shallower nanotextures preferentially decrease the reflectance at shorter λ ( Fig. 1e , blue colour), consistent with the requirement of t / λ >0.4 for full antireflection in a moth eye structure. Taller nanotextures extend the antireflection to longer λ ( Fig. 1e , red colour). We estimate n eff ( z ) for hexagonal arrangements of cones with subwavelength dimensions that taper to a point at their top ( z =0) and join at their base ( z = t ) using the effective medium approximation (EMA) ( q =0, Supplementary Methods ), valid for λ > π ·ℓ~200 nm, by calculating the fractional areal coverage of silicon [ f S ( z )] and air [ f A ( z )] versus depth ( z ): and f A ( z )=[1− f S ( z )]. Neglecting light absorption in air and silicon: with A and S are the frequency-dependent dielectric constants of air and silicon, respectively. The surface nanotexture provides broadband antireflection over a wide range of incident light angles. The reflectance of a flat silicon surface (at 650 nm) versus incident angle is markedly different for s- and p-polarized light, while a nanotextured silicon surface with t =230 nm and ℓ=52 nm displays similar, reduced reflectance for both polarizations ( Fig. 1f ). The texture’s deeply subwavelength lateral separation (ℓ) eliminates diffraction effects (that is, ℓ< λ /2 n for λ >400 nm), such that the average reflectance ( R ≡(spol+ppol)/2) remains <4% for angles as high as 60° from normal. The nanotexture provides omnidirectional antireflection across a broad λ -range. For example, at a 45° incident angle the average reflectance of s- and p-polarized light between 400 nm< λ <1 μm is <1%, more than 10 × smaller than that of flat silicon ( Fig. 1g ). Reflectance dependence on nanotexture dimensions Nanotextures made from self-assembled block copolymer templates with different ℓ have qualitatively similar vertical profiles and, when sufficiently tall, also provide high antireflection across a broad range of λ . A powerful characteristic of block copolymers as patterning materials is their lateral size tunability. For example, a cylindrical phase PS- b -PMMA with M w =67 kg mol −1 generates surface textures with ℓ=40±3 nm ( Fig. 2a ), while M w =132 and 177 kg mol −1 produce structures with ℓ=60±8 and 67±13 nm, respectively ( Fig. 2b ; Supplementary Fig. 2 ). Increasing the copolymer M w broadens the distributions of nearest neighbour separations (ℓ) ( Supplementary Fig. 3 ) and decreases the degree of hexagonal ordering ( Supplementary Fig. 4 ), because of slower self-assembly kinetics. However, neither of these affects the general results of our experiments because of the deeply subwavelength dimensions of our structures (ℓ ≪ λ ). 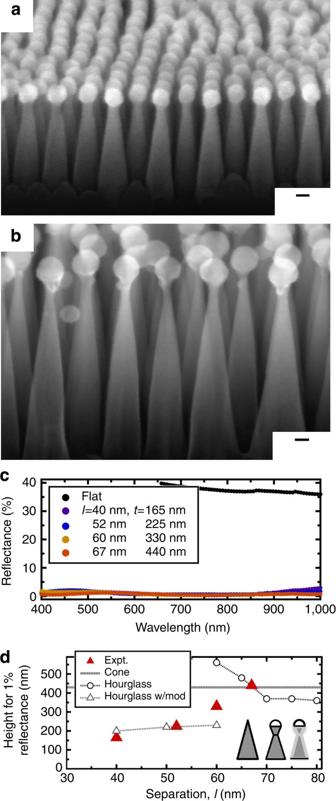Figure 2: Variation of antireflection performance with nanotexture separation. Scanning electron microscope (SEM) images (70°) of nanotextures made from (a) 67 kg mol−1polystyrene-b-poly(methyl methacrylate), witht=155 nm and ℓ=40 nm, and (b) 132 kg mol−1, witht=300 nm and ℓ=60 nm. Scale bar, 20 nm. (c) Measured reflectance versusλfor nanotextures with ℓ ranging from 40 to 67 nm, and correspondingtfrom 165 to 440 nm. (d) Measured height for 1% average broadband reflectance versus nanotexture separation, ℓ (red triangles). Transfer matrix calculations of the minimum height required for 1% average reflectance from (grey line) cone, (open circles) hourglass and (open triangles) hourglass with surface modification, versus nanotexture separation. The optical constants in surface modification calculations used values measured for ℓ=52 nm. (Inset) schematic nanotexture profiles. Figure 2: Variation of antireflection performance with nanotexture separation. Scanning electron microscope (SEM) images (70°) of nanotextures made from ( a ) 67 kg mol −1 polystyrene- b -poly(methyl methacrylate), with t =155 nm and ℓ=40 nm, and ( b ) 132 kg mol −1 , with t =300 nm and ℓ=60 nm. Scale bar, 20 nm. ( c ) Measured reflectance versus λ for nanotextures with ℓ ranging from 40 to 67 nm, and corresponding t from 165 to 440 nm. ( d ) Measured height for 1% average broadband reflectance versus nanotexture separation, ℓ (red triangles). Transfer matrix calculations of the minimum height required for 1% average reflectance from (grey line) cone, (open circles) hourglass and (open triangles) hourglass with surface modification, versus nanotexture separation. The optical constants in surface modification calculations used values measured for ℓ=52 nm. (Inset) schematic nanotexture profiles. Full size image Textures with smaller feature sizes outperform the geometric model of equation (1), needing <50% of the minimum height t ~0.4 × λ ~400 nm to achieve average broadband reflectance of <1%. The required nanotexture height decreases linearly with ℓ ( Fig. 2c ; Fig. 2d , red triangles), shrinking to only ~165 nm for ℓ=40 nm. The largest textures we measured (ℓ=67 nm) require a height of t =440 nm ( Fig. 2d , red triangles), similar to the value of 430 nm for <1% average reflectance calculated using the transfer matrix method ( Fig. 2d , grey line; Supplementary Methods ) and consistent with the taller heights of other silicon moth eye structures with larger lateral dimensions [12] , [14] , [27] . Calculations of the reflectance of a silicon nanotexture with an hourglass profile and alumina cap ( Fig. 2d , inset) also fail to capture the measured trend with decreasing ℓ ( Fig. 2d , open circles). Reflectance values calculated using the actual nanotexture refractive index profile measured by spectroscopic ellipsometry (SE) (for ℓ=52 nm) more accurately reproduce the measured data at smaller ℓ ( Fig. 2d , open triangles). Because the refractive index profile contains both shape- and material-dependent properties, we conclude that the measured reflectance results from combined effects of the geometry and modifications to the silicon surface optical properties ( Supplementary Fig. 9 ) [28] . The chlorine, bromine and oxygen etch chemistries we use to generate the nanotextures are known to modify the silicon within ~5–10 nm of the surface [28] , [29] , including redeposition of silicon oxychloride [30] , [31] , creating a surface layer with substantially different optical properties [32] and providing an additional mechanism for grading n i between air and silicon. In nanotextures with larger dimensions, this surface layer is an inconsequential fraction of the total volume. However, because our nanotextures have lateral feature sizes on the scale of 10 nm, even material modifications within a few nm of the surface comprise a significant volume fraction, and can thus substantially alter n i of the entire structure. We visualize changes in the nanotexture surface by comparing cross-sectional scanning electron microscope images before ( Fig. 3a ) and after ( Fig. 3b ) treating with a dilute (50:1) hydrofluoric acid:water mixture (buffered with NH 4 F), which removes surface oxides. In addition to stripping the alumina caps, the etch narrows the texture radius by several nm, consistent with removal of a silicon oxide layer that has been previously observed during studies of similar etch chemistries ( Supplementary Fig. 5 ) [30] , [31] . These results are consistent with transmission electron microscopy images showing the etched silicon nanotextures coated with an amorphous material ( Supplementary Fig. 6 ). X-ray photoelectron spectra of the nanotexture’s Si 2p and O 1s core levels display higher binding-energy peaks ( Supplementary Methods ; Supplementary Fig. 7 ), consistent with those of a material previously identified as a porous, anodic silicon oxide [33] . SE measurements of the complex refractive index profile ( n +i k ) of nanotextures with ℓ=52 nm and increasing t show the effect of such a modification, most easily observed at the nanotexture base, where n i increases abruptly from ~2 to the bulk silicon value ( n s =3.7) ( Fig. 3c ). In a two-dimensional close-packed arrangement of nanotextures composed of silicon alone, we would expect a n i reduced only slightly from that of silicon at the base ( n i ~3.5; equation (1) with z = t ). Transfer matrix reflectance calculations of silicon nanotextures (ℓ=52 nm) using optical constants obtained from SE measurements accurately describe the measured data for all nanotexture heights ( Fig. 3d ), capturing both the reflectance magnitude and optical resonance positions. These simulations provide a significantly improved description compared with similar calculations using bulk silicon optical constants ( Supplementary Fig. 9 ). 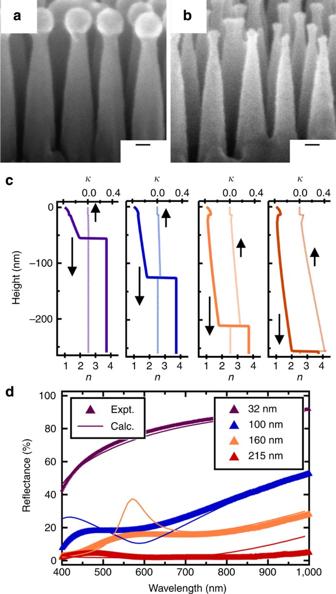Figure 3: Influence of a nanotexture refractive index profile. (a,b) 70° Angle scanning electron microscope (SEM) images of nanotextures (a) before and (b) after removal of surface oxide. Scale bar, 20 nm. (c) Spectroscopic ellipsometry measurements of the effective refractive index profile (n+iκ) at 750 nm wavelength for nanotextures with ℓ=52 nm and different heights. Up and down arrows refer plotted data to the appropriate horizontal axes. The procedure for obtaining these data is described in theSupplementary Methods. (d) Reflectance measurements (thick lines) and transfer matrix calculations (thin lines) (normalized to the flat substrate reflectance) versus wavelength for surface nanotextures with ℓ=52 nm and different heights. Geometric parameters used in the calculations are provided inSupplementary Table 1. Figure 3: Influence of a nanotexture refractive index profile. ( a,b ) 70° Angle scanning electron microscope (SEM) images of nanotextures ( a ) before and ( b ) after removal of surface oxide. Scale bar, 20 nm. ( c ) Spectroscopic ellipsometry measurements of the effective refractive index profile ( n +i κ ) at 750 nm wavelength for nanotextures with ℓ=52 nm and different heights. Up and down arrows refer plotted data to the appropriate horizontal axes. The procedure for obtaining these data is described in the Supplementary Methods . ( d ) Reflectance measurements (thick lines) and transfer matrix calculations (thin lines) (normalized to the flat substrate reflectance) versus wavelength for surface nanotextures with ℓ=52 nm and different heights. Geometric parameters used in the calculations are provided in Supplementary Table 1 . Full size image Applying the block copolymer-based surface nanotexture to a crystalline silicon solar cell improves the power conversion efficiency under AM1.5G illumination from 8.7 to 13.1% ( Fig. 4a ). The broadband antireflection improves the photocurrent ( J sc ) from 22 to 33 mA cm −2 , a substantial increase of 50% that agrees well with the integrated (from 400 to 1,000 nm) 50% increase in solar power transmitted to the device ( Supplementary Methods ; Supplementary Fig. 16 ). The photocurrent is significantly improved over that of similar planar devices coated instead with an optimized 80-nm-thick silicon nitride antireflection coating ( Fig. 4a , green open circles). The surface nanotexture allows the device to maintain nearly 100% of the J sc at normal incidence, even at oblique light angles 60° from normal ( Fig. 4b ). The performance of all three devices is limited by charge recombination, which manifests in the device dark current ( J 0 ) and diode ideality factor ( n diode ), and reduces the device open-circuit voltage ( V oc ). The silicon nitride antireflection coating slightly reduces both J 0 (to 10 −3 mA cm −2 ) and n diode (to ~1.8) compared with both planar and nanotextured devices (where J 0 ~3 × 10 −3 mA cm −2 and n diode ~2), which improves the device fill factor from 70 to 71%. Our future studies will target understanding the passivation effects of the nanotextured interface and integration with higher-performance devices. 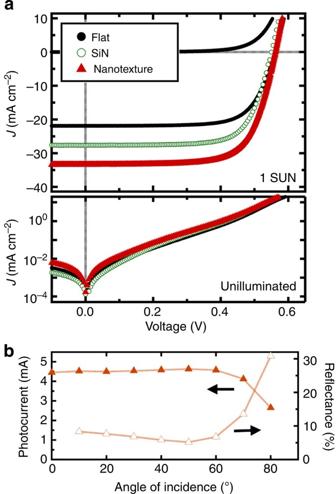Figure 4: Integration of nanotexture antireflection with silicon solar cells. (a) Illuminated (1 SUN) and unilluminated current–voltage (J–V) characteristics of (black) flat silicon solar cell and similar cells coated with (green open circles) an 80-nm-thick silicon nitride antireflection coating and (red) a surface nanotexture. (b) Angular dependence of device photocurrent (solid red triangles) and reflectance (red open triangles) when illuminated with 632-nm light. Left and right arrows refer plotted data to the appropriate horizontal axes. Figure 4: Integration of nanotexture antireflection with silicon solar cells. ( a ) Illuminated (1 SUN) and unilluminated current–voltage ( J – V ) characteristics of (black) flat silicon solar cell and similar cells coated with (green open circles) an 80-nm-thick silicon nitride antireflection coating and (red) a surface nanotexture. ( b ) Angular dependence of device photocurrent (solid red triangles) and reflectance (red open triangles) when illuminated with 632-nm light. Left and right arrows refer plotted data to the appropriate horizontal axes. Full size image Sample fabrication Our nanostructured samples included surface textures made from PS- b -PMMA block copolymers (Polymer Source Inc.) with molecular weights of M W =67 kg mol −1 (PS:PMMA 46:21, polydispersity PD=1.09), 99 kg mol −1 (PS:PMMA 64:35, PD=1.09), 132 kg mol −1 (PS:PMMA 96.5:35.5, PD=1.11) and 177 kg mol −1 (PS:PMMA 131:46, PD=1.10). We mixed solutions of all polymers in toluene at concentrations of 1% by weight. Block copolymer films were spin cast from solution onto silicon wafers at rates of 3K r.p.m. (67 K polymer), 2K r.p.m. (99 K polymer) and 1.6K r.p.m. (132 and 177 K polymers) and then annealed at <1 Torr at a temperature of 205 °C for 12 h. Prior to spin coating the block copolymer, we coated with a PS- r -PMMA random copolymer brush ( M W ≃ 11 kg mol −1 , PS:PMMA 52:48) by spin casting (0.4 wt % in toluene, 600 r.p.m. ), thermally annealing for 4 h and rinsing with toluene. We converted self-assembled PS- b -PMMA templates to aluminium oxide nanostructures by infiltration of the PMMA domains using three sequential exposures to tri-methyl aluminium and water vapour (for 300 s each at >5 Torr and 85 °C) in a commercial atomic layer deposition system (Cambridge Nanotech Savannah S100). We removed all remaining organic materials by oxygen plasma (20 W rf power, 100 mTorr O 2 , 2 min) using a March Plasma CS1701 etcher. We generate nanotextures in silicon having a conical profile by inductively coupled plasma-reactive ion etching using an Oxford Instrument Plasma Lab 100 with a 50:50:10 ratio of HBr, Cl 2 and O 2 gas (10 mTorr, 60 W rf power, 250 W inductive plasma power) at room temperature. We measure a vertical silicon etch rate of ~2 nm s −1 and a slower lateral etch rate of 0.07 nm s −1 . The process includes a 10-s breakthrough using BCl 3 and Cl 2 (20:5 standard cubic centimetre per minute, 10 mTorr, 100 W rf power, 800 W inductive plasma power). Samples were characterized by scanning electron microscopy (Hitachi S4800) operating at 20 kV. We fabricated silicon solar cells from Czochralski p-type (100) single-side-polished silicon wafers (550 μm thick, boron doped, 8 Ω cm). We used 4-cm 2 samples and are limited in our laboratory to 100-mm-diameter substrates. We formed the device p–n junction by diffusing phosphorous dopants from a solid source (ACCUSPIN, Honeywell P-8545) by first spin-coating at 3K r.p.m. for 30 s, baking on a hotplate at 150 °C (1 min) and annealing at 1,050 °C (20 s) in Ar using rapid thermal annealing processing. We removed the phosphosilicate glass from the substrate top surface using 10:1 buffered hydrofluoric acid (10 m). We formed the device back-contact by thermal evaporation of aluminium (100 nm) and annealing at 600 °C (1 m). The front-side contact was made with a photolithography-defined grid pattern and metal deposition of titanium (70 nm) and silver (100 nm). The total device area including front-side grid contacts is (0.5 cm) 2 . We deposited silicon nitride antireflection layers (80 nm) onto control devices by plasma-enhanced chemical vapour deposition prior to front- and back-contact metallization. We also formed surface nanotextures by the block copolymer process after p–n junction diffusion but prior to front- and back-contact metallization. Ultraviolet–visible light spectroscopy and spectroscopic ellipsometry We performed hemispherical reflectance measurements using a PerkinElmer Lambda 950 spectrophotometer equipped with an integrating sphere detector. The samples were placed at an 8° angle relative to the incident beam direction. Specular reflectivity for varying angle of incidence was measured using a supercontinuum laser at different wavelengths and angle of incidence ranging from 10° to 85°. We crosschecked these data with measurements using a Woollam Ellipsometer for angles of incidence >45°. We performed spectroscopic ellipsometry measurements using a J. A. Woollam Variable Angle Spectroscopic Ellipsometer M-2000, based on the diode array rotating compensator ellipsometer technology. We made measurements in three distinct spots on each sample in the wavelength range of 210–1,700 nm and at angles varying between 45° and 75° in divisions of 7.5°. We analysed ellipsometric data by simultaneously fitting identical models from each of the three spots, which were defined with coupled complex refractive indices, using the WVASE32 software (version 3.770, J. A. Woollam Co.). We determined the best fit for the optical constants by minimizing the mean square error between the measured and the modelled curves using the Levenberg–Marquardt multivariate regressions algorithm. We described the silicon material using a Drude model with critical-point-parabolic-band oscillators at 3.34 and 4.31 eV. Nanotextured silicon films were modelled using a graded EMA of optical constants of silicon and air/void, where the volume fraction of air/void versus depth is geometrically calculated. In this model, the optical constants determined from bare silicon were allowed to vary to give modified silicon optical constants. We divided the EMA layer into 40 slices and the modified silicon optical constants were held constant within each slice. More details can be found in the Supplementary Methods . X-ray photoelectron spectroscopy X-ray photoelectron spectroscopy measurements were performed in an ultrahigh vacuum system equipped with a SPECS Phoibos 100 hemispherical analyzer and a dual-anode X-ray source. All measurements were carried out with non-monochromatized Al Ka excitation. The measured data are fit with a Gaussian–Lorentzian product analysis (60% Lorentzian) carried out using CasaXPS software ( www.casaxps.com ). Optical modelling We computationally model the light reflection, transmission and absorption spectra by the different nanostructured surfaces using the transfer matrix method. For these calculations, we use the software package http://sjbyrnes.com/fresnel-solver.nb with some modifications. More details are provided in the Supplementary Methods . Solar cell measurement We measure the current–voltage characteristics of our silicon solar cells in the dark and under simulated AM1.5G illumination (calibrated using a certified silicon reference cell) at normal incidence using an HP4156B Semiconductor Parameter Analyzer. We perform the single-wavelength angular current–voltage measurements using a Thorlabs HNL150L EC, He Ne Laser at 632.8 nm. We mounted the sample on a Thorlabs CR1-Z7-motorized rotation stage and rotated in steps of 5°. The angular reflection measurements under oblique light incidence are carried out using a Fianium WL-Micro supercontinuum laser. The polarization of the incident light is selected using a Thorlabs broadband-polarizing beamsplitter cube and is adjusted using a half-wave plate. The incident/reflected light is detected using a Thorlabs PM100A power meter with a SV120VC silicon photo-detector. How to cite this article : Rahman, A. et al . Sub-50-nm self-assembled nanotextures for enhanced broadband antireflection in silicon solar cells. Nat. Commun. 6:5963 doi: 10.1038/ncomms6963 (2015).